Magnetoelectric control of frozen state in a toroidal glass The glass state of matter represents a frozen state of an atomically disordered system with local order only. Instead of atoms, systems with glassy states of magnetic and electric dipole moments in solids are known as spin and dipole glasses, respectively. In these conventional glasses, slow dynamics, such as relaxation and memory phenomena, are characteristics of their magnetic/dielectric properties. Here we propose a new glassy state in solids, a ‘toroidal glass’, in which toroidal moments—vector-like electromagnetic multipole moments breaking both space inversion and time reversal symmetries, and producing a linear magnetoelectric coupling—are randomly oriented and frozen. We investigate the dynamics of a linear magnetoelectric effect in Ni 0.4 Mn 0.6 TiO 3 and find that the magnetoelectric responses strongly depend on the magnetoelectric cooling history and show striking memory effects. These unusual magnetoelectric dynamical features can be explained in the framework of a toroidal glass in which the toroidal frozen state can be controlled magnetoelectrically. The magnetoelectric (ME) effect, that is, the induction of either magnetization M by an electric field E (ME E effect) or electric polarization P by a magnetic field H (ME H effect), is a sensitive probe of the magnetic symmetry of magnetic insulators [1] , [2] , [3] . The terms of the free energy F to be considered are F =− MH − PE − αHE – βHHE – γHEE …. Here the first and second terms are the Zeeman and Stark energies, respectively. The third and fourth (fifth) terms give the linear and quadratic ME effects in which P ( M ), linear or quadratic, in the applied field strength is induced by H ( E ), respectively. On the basis of symmetry analysis, the linear effect ( P = αH and M = αE with non-zero linear ME coefficient α ) is allowed only in magnetic insulators in which both space inversion and time reversal symmetries are broken. The toroidal moment t can be generated either by persistent orbital currents or certain spin orderings [4] , [5] . In the latter case, t is known as a multi-spin variable breaking both space inversion and time reversal symmetries, and is defined as t Σ i r i × S i , where r i denotes the location of spin S i (refs 4 , 5 ). When t is non-zero, an off-diagonal and antisymmetric linear ME effect is allowed, that is, P − t × H and M t × E , which are obtained from the free energy expansion analysis [6] , [7] . Thus, magnetic insulators showing a ferrotoroidic order (for example, Ga 2- x Fe x O 3 and LiCoPO 4 ) can exhibit the antisymmetric linear ME effect [8] , [9] , [10] . Recently, an XY -like spin glass Ni x Mn 1- x TiO 3 ( x ≈0.42) [11] , [12] was found to show the off-diagonal and antisymmetric linear ME H effect [13] , although a linear ME effect is rarely seen in magnetically disordered systems, such as spin glasses. (A higher-order ME effect is seen in perovskite (Sr,Mn)TiO 3 , so-called ‘multiglass’, in which dipole and spin glass states coexist [14] .) In Ni x Mn 1- x TiO 3 with the ilmenite structure (centrosymmetric space group R ), a magnetic (Ni,Mn) plane and a non-magnetic Ti plane are alternately stacked along the hexagonal c axis. The Ni 2+ and Mn 2+ ions are randomly distributed in the (Ni,Mn) plane and form a honeycomb lattice (inset of Fig. 1b ). Ni 0.4 Mn 0.6 TiO 3 (hereafter NMTO) exhibits successive spin glass transitions at T SG1 ≈9.5 K and T SG2 ≈6 K [11] , [13] , and is classified as an XY -like spin glass with an easy-plane anisotropy [15] . The recently discovered antisymmetric linear ME H effect in NMTO possesses ME tensor components α 12 =− α 21 ≠0 below about 9 K [13] . The ME H effect was reasonably explained by considering that the presence of the cross-product of E and H , ( E × H ), during the spin-freezing process polarizes net t in the direction perpendicular to the honeycomb lattices. Thus, NMTO is a rare example showing that disordered frozen spins purely induce a linear ME coupling. This study examines cooling history and dynamical features, which are the most intriguing characteristics of the glassy frozen states, in the ME effect of NMTO and provide a new concept, ‘toroidal glass’. 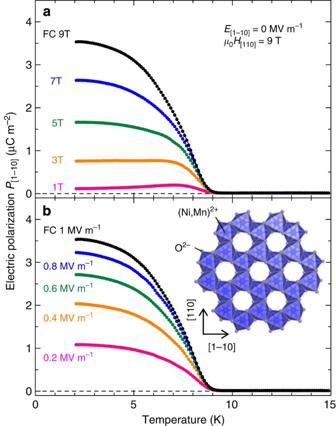Figure 1:ME-cooling-condition dependence onPinduced by MEHeffect in NMTO. Tdependence ofP[1–10]measured atμ0H[110]=9 T andE[1–10]=0 MV m−1after several ME cooling procedures (a) at fixedE[1–10]=1 MV m−1and variousμ0H[110]from 1 to 9 T (b) at variousE[1–10]from 0.2 to 1 MV m−1andμ0H[110]=9 T. (For example, ‘FC 1 MV m−1’ denotes the data ME-cooled atE[1–10]=1 MV m−1.) Inset ofb, crystal structure of NMTO projected along the hexagonalcaxis. Randomly distributed Ni2+and Mn2+ions form stacked honeycomb lattices. Figure 1: ME-cooling-condition dependence on P induced by ME H effect in NMTO. T dependence of P [1–10] measured at μ 0 H [110] =9 T and E [1–10] =0 MV m −1 after several ME cooling procedures ( a ) at fixed E [1–10] =1 MV m −1 and various μ 0 H [110] from 1 to 9 T ( b ) at various E [1–10] from 0.2 to 1 MV m −1 and μ 0 H [110] =9 T. (For example, ‘FC 1 MV m −1 ’ denotes the data ME-cooled at E [1–10] =1 MV m −1 .) Inset of b , crystal structure of NMTO projected along the hexagonal c axis. Randomly distributed Ni 2+ and Mn 2+ ions form stacked honeycomb lattices. Full size image Cooling-condition dependence of ME effect First, we examine the ME-cooling-condition dependence on P induced by the ME H effect in a single crystal of NMTO. Figure 1 shows temperature ( T ) profiles of P parallel to the [1–10] direction ( P [1–10] ) at μ 0 H =9 T along [110] ( H [110] ). This configuration allows measurement of the ME tensor components α 12 (or α 21 ). Before the respective measurements, the specimen was cooled from 20 K (> T SG1 ) to 2 K in finite | E × H | with selected E along [1–10] ( E [1–10] ) and H [110] (ME field cooling). Then, P [1–10] was taken at μ 0 H [110] =9 T in the absence of E [1–10] . All the data shown in Fig. 1a were taken after ME field cooling with E [1–10] =1 MV m −1 and selected H [110] . Below 9 K, magnetoelectrically induced P [1–10] develops in all the data. It is noteworthy that the magnitude of P [1–10] strongly depends on the strength of cooling H [110] . Figure 1a clearly demonstrates that P [1–10] monotonically increases with increasing the cooling H [110] . We also measured the cooling E dependence of P [1–10] . The results are shown in Fig. 1b . Before these measurements, μ 0 H [110] =9 T and selected E [1–10] were applied during the ME-field-cooling process. The magnitude of P [1–10] monotonously increases as the cooling E [1–10] increases. These results indicate that the magnitude of P is very sensitive to both cooling E and H , that is, ME-field-cooling condition. The observed remarkable cooling H and E effects on P are reminiscent of the cooling H effect on M in spin glasses [16] and/or the cooling E effect on P in dipole glasses [17] . In ref. 13 , it was proposed that the ME H effect, that is, the induction of P [1–10] by applying H [110] , observed in NMTO originates from the presence of net toroidal moment t along [001] through the relation P − t × H . If this scenario is correct, we can also expect the ME E effect, the induction of M along [110] ( M [110] ) induced by applying E [1–10] , with the relation M t × E from phenomenological consideration [7] . Thus, we examined the ME E effect in NMTO. 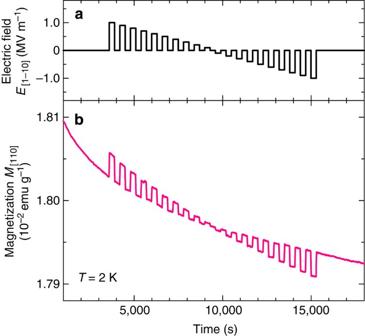Figure 2:Relaxation ofMand MEEeffect in NMTO. Temporal evolution of (b) isothermalM[110]responding to (a) periodically appliedE[1–10]atT=2 K andμ0H[110]=0 T. Before the measurement, ME cooling was done withμ0H[110]=7 T andE[1–10]=1 MV m−1. Figure 2b shows the time dependence of M [110] at μ 0 H [110] =0 T and T =2 K. Before the measurement, the ME cooling procedure was done with μ 0 H [110] =7 T and E [1–10] =1 MV m −1 . As is common with spin glasses, a remnant magnetization caused by the magnetic-field cooling appears and shows a long-time relaxation [16] . During the relaxation process, various strengths of E [1–10] were applied, as plotted in Fig. 2a . Comparing Fig. 2a it is evident that the magnitude of M [110] systematically changes, depending on the strength and sign of applied E [1–10] . Such an effect of E [1–10] on M [110] was not observed without the ME-field-cooling process. This result clearly confirms the presence of the ME E effect in NMTO. Figure 2: Relaxation of M and ME E effect in NMTO. Temporal evolution of ( b ) isothermal M [110] responding to ( a ) periodically applied E [1–10] at T =2 K and μ 0 H [110] =0 T. Before the measurement, ME cooling was done with μ 0 H [110] =7 T and E [1–10] =1 MV m −1 . 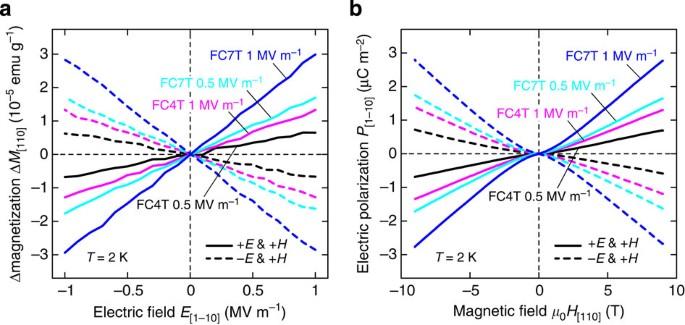Figure 3:Comparison of MEEand MEHeffect in NMTO. (a)E[1–10]dependence of ΔM[110]=M[110](E)−M[110](0) and (b)H[110]dependence ofP[1–10]atT=2 K after ME cooling with selectedE[1–10]andH[110]. (For example, ‘FC7T 1 MV m−1, denotes the data ME-cooled atμ0H[110]=7 T andE[1–10]=1 MV m−1.) Solid and broken lines represent the data taken after ME cooling with (+E, +H) and (–E, +H), respectively. Full size image Figure 3a displays E [1–10] profiles of the change in remanent magnetization [Δ M [110] = M [110] ( E )− M [110] (0)] measured at μ 0 H [110] =0 T and T =2 K. Before each measurement, the ME-field cooling was performed at various E [1–10] and H [110] . As seen in Fig. 3a , Δ M [110] shows the linear E [1–10] dependence, Δ M [110] = α m E [1–10] , and the sign of α m is reversed by changing the sign of the ME field ( E × H ) upon cooling. (Compare solid and broken lines in the same colour.) In addition to the linear E dependence, the magnitude of Δ M [110] (or α m ) strongly depends on that of ( E × H ) upon cooling. As | E × H | increases, α m monotonically increases. To compare the ME E effect with the ME H effect, we also show in Fig. 3b the H [110] dependence of P [1–10] measured at E [1–10] =0 MV m −1 and T =2 K after the selected preparatory ME cooling procedures. As seen in Fig. 3a , the ME H and ME E effects show a similar ME-field-cooling dependence. The ME coefficient α p (= dP/dH ) obtained from the P–H curve cooled at μ 0 H [110] =7 T and E [1–10] =1 MV m −1 is ~0.2 ps m −1 at around 0 T. Meanwhile, α m obtained from the M–E curve for the same ME-field-cooling condition is ~0.2 ps m −1 . This good agreement indicates that the origin of the ME H and ME E effects is the same, and supports the presence of net t [13] . Figure 3: Comparison of ME E and ME H effect in NMTO. ( a ) E [1–10] dependence of Δ M [110] = M [110] ( E )− M [110] (0) and ( b ) H [110] dependence of P [1–10] at T =2 K after ME cooling with selected E [1–10] and H [110] . (For example, ‘FC7T 1 MV m −1 , denotes the data ME-cooled at μ 0 H [110] =7 T and E [1–10] =1 MV m −1 .) Solid and broken lines represent the data taken after ME cooling with (+ E , + H ) and (– E , + H ), respectively. Full size image ME memory effect We also found that NMTO shows the ME version of ‘memory effect’, which is common in glassy systems [18] , [19] , [20] , [21] . First, we took P [1–10] by a usual measurement process: P [1–10] was taken upon warming at μ 0 H [110] =9 T and E [1–10] =0 MV m −1 after ME cooling at μ 0 H [110] =9 T and E [1–10] =1 MV m −1 . The obtained P [1–10] is referred to as the reference curve ( P ref ) (a black solid curve in Fig. 4a ). Then, we again measured P [1–10] by the same procedure, except for including a halt for t h =3,600 s at an intermediate temperature T h (=6 K or 5 K) during cooling. During the halt, E [1–10] was turned off. The schematic measurement protocol is illustrated in the inset of Fig. 4b . For all the measurements, the cooling and warming rate is constant at 1 K min −1 . As seen in Fig. 4a , P [1–10] after a halt on cooling ( P h ) slightly decreases compared with P ref below T h . A more distinct difference is observed in between − dP ref / dT and − dP h / dT (see Fig. 4b ). The T dependence of − dP h / dT with T h =6 K shows a ‘dip’-like structure around T h =6 K, and − dP h / dT almost overlaps − dP ref / dT below 5.5 K and above 7 K. In the data of T h =5 K, − dP h / dT clearly shows a dip around T h =5 K. We also measured t h dependence of P [1–10] . As seen in Fig. 4c , P [1–10] measured at 5 K for T h =6 K shows a slow decay over t h =1 h. These results clearly indicate that the long-time relaxation of P [1–10] occurs during the halts and NMTO memorizes the halt during cooling. Thus, we successfully observed the slow dynamics and memory effect by use of ME effect for the first time. 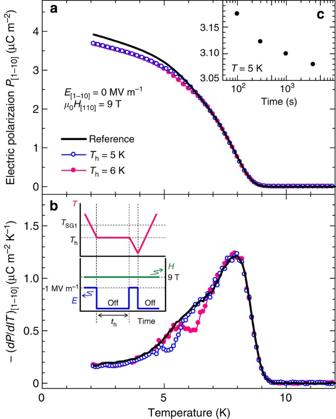Figure 4: ME memory effect in NMTO. Temperature dependence of (a)P[1–10]and (b) −(dP/dT)[1–10]taken upon warming atμ0H[110]=9 T andE[1–10]=0 MV m−1. The solid black line shows a reference curve taken after continuous field cooling atμ0H[110]=9 T andE[1–10]=1 MV m−1. The open blue circles and closed red circles were measured after a halt atTh=5 K and 6 K, respectively, during the same field-cooling procedure. During the halt time,E[1–10]was turned off. (c) Thethdependence ofP[1–10]measured at 5 K forTh=6 K. Inset ofb, schematic representation of field-cooling and warming procedure, including a halt. The upper panel shows the temporal evolution ofT, and the lower panel shows those ofEandHduring a ME cooling and a measurement. Figure 4: ME memory effect in NMTO. Temperature dependence of ( a ) P [1–10] and ( b ) −( dP / dT ) [1–10] taken upon warming at μ 0 H [110] =9 T and E [1–10] =0 MV m −1 . The solid black line shows a reference curve taken after continuous field cooling at μ 0 H [110] =9 T and E [1–10] =1 MV m −1 . The open blue circles and closed red circles were measured after a halt at T h =5 K and 6 K, respectively, during the same field-cooling procedure. During the halt time, E [1–10] was turned off. ( c ) The t h dependence of P [1–10] measured at 5 K for T h =6 K. Inset of b , schematic representation of field-cooling and warming procedure, including a halt. The upper panel shows the temporal evolution of T , and the lower panel shows those of E and H during a ME cooling and a measurement. Full size image Let us discuss the cooling-( E × H ) dependence of the ME effect in NMTO. According to the consideration of the free energy in a magnetic system in which spin ordering breaks the time reversal and space inversion symmetries, the free energy related to the ME effect is expressed as F ME =– a ( E · H ) – t · [ E × H ] …, where the pseudoscalar a is coupled to the divergence of magnetic field, and is zero in the absence of magnetic monopoles [7] . This means that the free energy is stabilized by the presence of ( E × H ) and a toroidal moment t along ( E × H ). Meanwhile, in spin glass systems with replica symmetry breaking [22] , multi-valley structures in their free energies are considered to develop and be responsible for their characteristics, such as slow relaxations, dependence on initial conditions and remanent effects. Thus, it is reasonable to consider that one of the multi-valley states having net t is stabilized due to the presence of a certain ( E × H ) during the spin-freezing process and that the change in the magnitude of ( E × H ) during the freezing makes the system into a different valley state with a different net t . 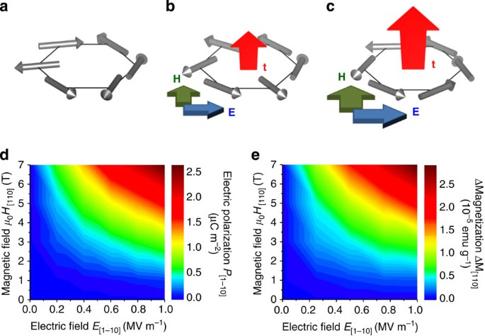Figure 5: Toroidal frozen state controlled magnetoelectrically. (a–c) Proposed relationships among the strength of ME cooling field (E×H), the induced spin (gray arrow) configurations and the concomitant toroidal momenttin the spin-frozen state for NMTO with the honeycomb lattice. (d) Contour plot ofP[1–10]measured atT=2 K,μ0H[110]=9 T, andE[1–10]=0 MV m−1versusE[1–10]andH[110]upon the ME-field-cooling process. (e) Counter plot of ΔM[110]atT=2 K,μ0H[110]=0 T, andE[1–10]=1 MV m−1versusE[1–10]andH[110]upon ME-field-cooling process. Figure 5a–c depicts proposed schematic spin configurations of the spin-frozen states after ME cooling processes at zero, low and high ME fields ( E × H ), respectively. Free energy related with toroidal moment t can be expressed as F t =− t · ( E × H ) [7] . Thus, when | E × H | is absent upon cooling, there is no energy gain by the presence of t , and then no net t develops, which means spins with an easy-plane anisotropy are randomly oriented within the plane ( Fig. 5a ). However, by cooling the system in the finite ME fields | E × H |, the induction of net t gives rise to energy gain ( Fig. 5b ). As | E × H | upon cooling increases, freezing spins are gradually oriented in a vortex-like manner, each local t polarized along the same direction, and then net t increases ( Fig. 5c ). This scenario well explains the observed ME-field-cooling dependence of ME E and ME H effects ( Fig. 3 ). Figure 5d display contour plots of the magnitude of P [1–10] and Δ M [110] versus the strength of E [1–10] and H [110] upon cooling, respectively. Both Δ M [110] and P [1–10] , that is, α m and α p , monotonically increase with increasing | E × H |. These plots further confirm the above scenario and demonstrate ME control of the spin-frozen state (or net t ) by changing | E × H |. In addition, the observed ME-field-cooling dependence indicates that there are a number of metastable toroidal frozen states. Such huge degeneracy is discussed as the multi-valley structure in free energy for conventional spin glasses with replica symmetry breaking [22] and can be observed as the cooling H dependence of M [16] , [23] . In other words, toroidal moments in NMTO appear to behave as glass. Furthermore, the ME slow dynamics, as observed for the memory effect, strongly suggest the validity of the glass nature of toroidal moment. Figure 5: Toroidal frozen state controlled magnetoelectrically. ( a – c ) Proposed relationships among the strength of ME cooling field ( E × H ), the induced spin (gray arrow) configurations and the concomitant toroidal moment t in the spin-frozen state for NMTO with the honeycomb lattice. ( d ) Contour plot of P [1–10] measured at T =2 K, μ 0 H [110] =9 T, and E [1–10] =0 MV m −1 versus E [1–10] and H [110] upon the ME-field-cooling process. ( e ) Counter plot of Δ M [110] at T =2 K, μ 0 H [110] =0 T, and E [1–10] =1 MV m −1 versus E [1–10] and H [110] upon ME-field-cooling process. Full size image When looking at the above-mentioned ME-related free energy F ME , the development of net the pseudoscalar a , which is related to magnetic monopoles, can also be expected in the presence of ( E · H ). However, we did not observe any ME signals after the ME-field-cooling only with finite ( E · H ). Hence, such a spin-frozen state may not exist in the present system, although we do not have a clear reason at this time. Thus, we conclude that there exists a novel glass state in solids, termed ‘toroidal glass’, which is regarded as the glass of the fourth ordered form, ‘(anti)ferrotoroidic ordered state’ [6] , [7] . Measurements of ME-cooling-condition dependence of magnetochiral dichroism, non-reciprocal X-ray gyrotropy and magnetic diffuse scattering can be other complementary methods to verify the toroidal glass state [7] , [24] . Other XY -like spin glass systems (for example, BaCo 6 Ti 6 O 19 (ref. 25 )) can be promising candidates having the toroidal glass state. Crystal growth A single crystal of NMTO was grown by the floating zone method, as reported previously [26] . First, a polycrystalline feed rod was prepared by a solid-state reaction. Stoichiometric quantities of NiO, Mn 3 O 4 and TiO 2 powders with 99.9% purity were mixed and heated at 1,000 °C for 10 h in air. The resulting polycrystalline sample was ground into powders again, and then pressed into a rod with the dimension of about 6 mm in diameter and 100 mm in length. The rod was sintered again at 1,100 °C for 15 h in air. The crystal growth was carried out on the sintered rod with the use of a halogen-lamp image furnace in flowing air at a rate of 500 ml min −1 . The growth rate was 1–3 mm h −1 . Thus, a single crystal with clear facets parallel to the c -plane (hexagonal setting) was obtained. Measurements of ME effects The obtained crystal was oriented with use of Laue X-ray diffraction patterns and was cut into two rectangular plates with the widest faces parallel to the (1–10) plane. The dimensions of these specimens were 17.5 mm 2 × 0.1 mm and 18.5 mm 2 × 0.4 mm for measurements of electric polarization ( P ) and magnetization ( M ), respectively. Silver electrodes were vacuum-deposited onto the widest faces of these specimens. To obtain P parallel to [1–10] ( P [1–10] ) as functions of temperature ( T ) and magnetic field ( H ) applied along [110] ( H [110] ), pyroelectric and ME currents were measured during T - and H -sweeping procedures, respectively, in a superconducting magnet (Quantum Design, PPMS) by using an electrometer (Keithley Instruments 6517A). To measure M along [110] ( M [110] ) as a function of electric field ( E ) applied along [1–10] ( E [1–10] ), a home-made insert, which allows the application of E during M measurements was installed in a magnetometer (Quantum Design, MPMS SQUID VSM). On the home-made insert, the silver electrodes vacuum-deposited onto the sample were electrically connected with an external voltage source (Keithley Instruments 6517A) via copper wires. All the ME measurements were done after ME-field-cooling procedures at selected E [1–10] and H [110] . How to cite this article: Yamaguchi, Y. & Kimura, T. Magnetoelectric control of frozen state in a toroidal glass. Nat. Commun. 4:2063 doi: 10.1038/ncomms3063 (2013).